Error-corrected quantum annealing with hundreds of qubits Quantum information processing offers dramatic speedups, yet is susceptible to decoherence, whereby quantum superpositions decay into mutually exclusive classical alternatives, thus robbing quantum computers of their power. This makes the development of quantum error correction an essential aspect of quantum computing. So far, little is known about protection against decoherence for quantum annealing, a computational paradigm aiming to exploit ground-state quantum dynamics to solve optimization problems more rapidly than is possible classically. Here we develop error correction for quantum annealing and experimentally demonstrate it using antiferromagnetic chains with up to 344 superconducting flux qubits in processors that have recently been shown to physically implement programmable quantum annealing. We demonstrate a substantial improvement over the performance of the processors in the absence of error correction. These results pave the way towards large-scale noise-protected adiabatic quantum optimization devices, although a threshold theorem such as has been established in the circuit model of quantum computing remains elusive. Combinatorial optimization problems are of great interest in both complexity theory and practical applications, and are also notoriously difficult to solve [1] . Quantum computing harbours the promise of dramatic speedups over its classical counterpart [2] , yet it cannot function on a large scale without error correction [3] . Quantum annealing, a form of quantum computing tailored to optimization that can be more efficient than classical optimization [4] , [5] , [6] , also requires error correction. Quantum annealing is an alternative to classical simulated annealing, an approach to optimization based on the observation that the cost function of an optimization problem can be viewed as the energy of a physical system, and that energy barriers can be crossed by thermal hopping [7] . However, to escape local minima it can be advantageous to explore low-energy configurations quantum mechanically by exploiting superpositions and tunnelling. Quantum annealing is based on this idea and was originally introduced as an algorithm designed to solve optimization problems such as minimizing multidimensional functions [8] or finding the ground states of classical spin Hamiltonians [9] . Quantum annealing is closely related to adiabatic quantum computation [10] , [11] , a paradigm that is computationally universal (hence, not limited to optimization) and is equivalent in computational power to the standard circuit model of quantum computation up to polynomial overhead [12] , [13] . The physical realization of the quantum annealing algorithm [14] , [15] , [16] , [17] is called a programmable quantum annealer (PQA). Numerous experiments have demonstrated the utility of quantum error correction in gate-model quantum computing with up to nine qubits using, for example, NMR [18] , [19] , trapped ions [20] , [21] , optical systems [22] , [23] and superconducting circuits [24] . However, such demonstrations require far more control than is available in PQA. Similarly, most error correction or suppression methods developed for adiabatic quantum computing [25] , [26] , [27] , [28] beyond a classical repetition code [16] require operations that are not included in the PQA repertoire. Furthermore, an accuracy-threshold theorem, such as exists for circuit model quantum computing [29] , [30] , [31] , is still lacking for adiabatic quantum computing. Thus, it remains an open theoretical question whether a noisy PQA can accurately simulate an ideal PQA for arbitrary large optimization problems. In spite of these obstructions, here we develop and demonstrate an error correction method for PQA. This method can improve the success probability of quantum annealing, while full-fledged fault tolerance remains an open problem. We provide an experimental demonstration using up to 344 superconducting flux qubits in D-Wave processors [17] , [32] , which have recently been shown to physically implement PQA [33] , [34] , [35] , [36] , [37] . At this time, there is no conclusive evidence that the D-Wave processors can outperform the best classical algorithms, and the question remains the subject of considerable debate [38] , [39] . The qubit connectivity graph of these processors is depicted in Fig. 1a . 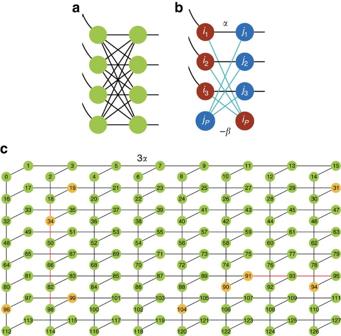Figure 1: Unit cell and encoded graph. (a) Schematic of one of the 64 unit cells of the DW2 processor; unit cells are arranged in an 8 × 8 array forming a ‘Chimera’ graph between qubits (see Methods). Each circle represents a physical qubit and each line a programmable Ising coupling. Lines on the right (left) couple to the corresponding qubits in the neighbouring unit cell to the right (above). (b) Two ‘logical qubits’ (i, red andj, blue) embedded within a single unit cell. Qubits labelled 1–3 are the ‘problem qubits’, the opposing qubit of the same colour labelledPis the ‘penalty qubit’. Problem qubits couple via the black lines with tunable strengthαboth inter- and intraunit cell. Light blue lines of magnitudeβare ferromagnetic couplings between the problem qubits and their penalty qubit. (c) Encoded processor graph obtained from the Chimera graph by replacing each logical qubit by a circle. This is a non-planar graph (see Methods for a proof) with couplings of strength 3α. Green circles represent complete logical qubits. Orange circles represent logical qubits lacking their penalty qubit (see Methods). Red lines are groups of couplers that cannot all be simultaneously activated. Figure 1: Unit cell and encoded graph. ( a ) Schematic of one of the 64 unit cells of the DW2 processor; unit cells are arranged in an 8 × 8 array forming a ‘Chimera’ graph between qubits (see Methods). Each circle represents a physical qubit and each line a programmable Ising coupling . Lines on the right (left) couple to the corresponding qubits in the neighbouring unit cell to the right (above). ( b ) Two ‘logical qubits’ ( i , red and j , blue) embedded within a single unit cell. Qubits labelled 1–3 are the ‘problem qubits’, the opposing qubit of the same colour labelled P is the ‘penalty qubit’. Problem qubits couple via the black lines with tunable strength α both inter- and intraunit cell. Light blue lines of magnitude β are ferromagnetic couplings between the problem qubits and their penalty qubit. ( c ) Encoded processor graph obtained from the Chimera graph by replacing each logical qubit by a circle. This is a non-planar graph (see Methods for a proof) with couplings of strength 3 α . Green circles represent complete logical qubits. Orange circles represent logical qubits lacking their penalty qubit (see Methods). Red lines are groups of couplers that cannot all be simultaneously activated. Full size image Quantum annealing and computational errors Many hard and important optimization problems can be encoded into the lowest energy configuration (ground state) of an Ising Hamiltonian where each σ i z =±1 is a classical binary variable, and the dimensionless local fields h :={ h i } and couplings J :={ J ij } are the ‘programmable’ parameters that specify the problem [40] , [41] . In PQA the solution of the optimization problem is found by replacing the classical variables by N quantum binary variables (qubits) that evolve subject to the time-dependent Hamiltonian Here H X = is a transverse-field Hamiltonian, and denote the spin 1/2 Pauli operators whose eigenstates are, respectively, |0〉, |1〉 and |±〉=(|0〉±|1〉)/ , with eigenvalues ±1. A ( t ) and B ( t ) are time-dependent functions (with dimensions of energy) satisfying A ( t f )= B (0)=0, and t f is the annealing time. A physical PQA always operates in the presence of a thermal environment at temperature T . Provided A (0) ≫ k B T , the PQA is initialized in the ground state of H X , namely, the uniform superposition state (|0 ⋯ 0〉 + ⋯ + |1 ⋯ 1〉)/ . Provided B ( t f ) ≫ k B T , the final state at the end of the annealing process is stable against thermal excitations when it is measured. If the evolution is adiabatic, that is, if H ( t ) is a smooth function of time and if the gap Δ:= ε 1 ( t )−ε 0 ( t ) between the first excited-state energy ε 1 ( t ) and the ground-state energy ε 0 ( t ) is sufficiently large compared with both 1/ t f and T , then the adiabatic approximation for open systems [42] , [43] , [44] , [45] guarantees that the desired ground state of H Ising will be reached with high fidelity at t f . However, hard problems are characterized by gaps that close superpolynomially or even exponentially with increasing problem size [10] , [11] , [46] . If the gap is too small, then both non-adiabatic transitions and thermal excitations can result in computational errors, manifested in the appearance of excited states at t f . While the non-adiabatic transition rate can in principle be suppressed to an arbitrarily high degree by enforcing a smoothness condition on the annealing functions A ( t ) and B ( t ) [47] , thermal excitations will cause errors at any non-zero temperature. In addition, even if Δ is large enough, inaccuracies in the implementation of H Ising may result in the evolution ending up in the ‘wrong’ ground state. Overcoming such errors requires error correction. Quantum annealing correction We devise a strategy we call ‘quantum annealing correction’ (QAC), comprising the introduction of an energy penalty (EP) along with encoding and error correction. Our main tool is the ability to independently control pairwise Ising interactions, which can be viewed as the generators of the bit-flip stabilizer code [48] . We first encode H Ising , replacing each term by its encoded counterpart and each by , where the subindices ℓ refer to the problem qubits as depicted in Fig. 1b . After these replacements we obtain an encoded Ising Hamiltonian where is the number of encoded qubits. This encoding allows for protection against bit-flip errors in two ways. First, the overall problem energy scale is increased by a factor of n , where n =3 in our implementation on the D-Wave processors. Note that since we cannot also encode H X (this would require n -body interactions), it does not directly follow that the gap energy scale also increases; we later present numerical evidence that this is the case, so that thermal excitations will be suppressed. Second, the excited-state spectrum has been labelled in a manner that can be decoded by performing a post-read-out majority vote on each set of n problem qubits, thereby error-correcting non-code states into code states to recover some of the excited-state population. The ( n , 1) repetition code has minimum Hamming distance n , that is, a non-code state with more than ⌊ n /2 ⌋ bit-flip errors will be incorrectly decoded; we call such states ‘undecodable’, while ‘decodable states’ are those excited states that are decoded via majority vote to the correct code state (see Methods for details of the code and non-code states). To generate additional protection, we next introduce a ferromagnetic penalty term the sum of stabilizer generators of the n +1 qubit repetition code, which together detect and energetically penalize [25] all bit-flip errors except the full encoded qubit flip. The role of H P can also be understood as to lock the problem qubits into agreement with the penalty qubit, reducing the probability of excitations from the code space into non-code states; see Fig. 1b for the D-Wave processor implementation of this penalty. The encoded graph thus obtained in our experimental implementation is depicted in Fig. 1c . Including the penalty term, the total encoded Hamiltonian we implement is where + β H P , and the two controllable parameters α and β are the ‘problem scale’ and ‘penalty scale’, respectively, which we can tune between 0 and 1 in our experiments and optimize. Note that our scheme, as embodied in equation (5), implements QAC: H P energetically penalizes every error E it does not commute with, for example, every single-qubit error E ε U (2) such that E σ z . To illustrate this, consider the case where E = . Early in the quantum annealing evolution when the transverse-field Hamiltonian dominates, such an error corresponds to a phase-flip error, while late in the evolution when the Ising Hamiltonian dominates it is a bit-flip error. Denoting the instantaneous ground state of the total encoded Hamiltonian minus the penalty term, , by and the ‘erred’ state by (either another ground state or an excited state of ), the instantaneous energy difference between the erred state and the ground state is , where and . Thus, the EP will suppress thermal excitations from the ground state to the erred state except early in the evolution when B ( t )=0. In contrast, an error that commutes with the penalty term, such as any pure phase-flip error , is not penalized. Benchmarking using antiferromagnetic chains Having specified the general scheme, which in particular is applicable to any problem that is embeddable on the encoded graph shown in Fig. 1c , we now focus on antiferromagnetic chains. In this case, the classical ground states at t = t f are simply the doubly degenerate states of nearest-neighbour spins pointing in opposite directions. This allows us to benchmark our QAC strategy while focusing on the role of the controllable parameters, instead of the complications associated with the ground states of frustrated Ising models [35] , [49] . Moreover, chains are dominated by domain wall errors [17] , which as we explain below are a particularly challenging scenario for our QAC strategy. As a reference problem, we implemented an N -qubit antiferromagnetic chain with H Ising ( α )= α . We call this problem ‘unprotected’ (U) since it involves no encoding or penalty. We can augment the U strategy by implementing four unpenalized parallel N -qubit chains: . We can decode the parallel chains in two ways. The first, which is our best classical alternative approach (C), treats the parallel chains as independent runs. If the chains are independent, this increases the success probability from p for the U strategy to 1−(1− p ) 4 for the C strategy. As shown in Fig. 2 , this prediction is in good overall agreement with our experimental results, with small deviations (probably due to crosstalk) appearing only for the longest chains. The binomial theory always gives an upper bound on the experimental results, suggesting that deviations from theory may be attributable to correlated errors in the experimental device. 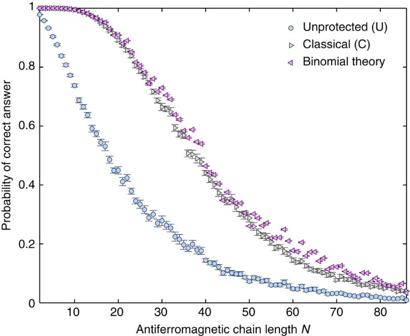Figure 2: Unprotected chains and the classical decoding strategy. Shown is a comparison of the experimental U and C results for chains of lengthN, along with the binomial theory prediction 1−(1−p)4, for problem scaleα=0.3. The U series is the input for the binomial theory. Here and in all subsequent figures error bars are calculated over the set of embeddings and express the s.e.m.σ/, whereσ2=is the sample variance andS=5,000 is the number of samples. Figure 2: Unprotected chains and the classical decoding strategy. Shown is a comparison of the experimental U and C results for chains of length N , along with the binomial theory prediction 1−(1− p ) 4 , for problem scale α =0.3. The U series is the input for the binomial theory. Here and in all subsequent figures error bars are calculated over the set of embeddings and express the s.e.m. σ / , where σ 2 = is the sample variance and S =5,000 is the number of samples. Full size image The second decoding strategy is to treat each triple of bits as an encoded bit i , which is decoded via majority vote. We call this the ‘no penalty’ (NP) strategy since it is the QAC strategy with β =0. As a third reference problem, we implemented a chain of -encoded qubits with an EP: . When we add majority vote decoding to the EP strategy we have our complete QAC strategy. Comparing the probability of finding the ground state in the U, C, NP, EP and QAC cases allows us to isolate the effects of the various components of the error correction strategy. As antiferromagnetic chains have two degenerate ground states, below we consider the ground state for any given experimentally measured state to be that with which the majority of the decoded qubits align. Experimental success probabilities The performance of the different strategies is shown in Fig. 3 . Our key finding is the high success probability of the complete QAC strategy for α =1 ( Fig. 3a ), improving significantly over the four other strategies as the chain length increases, and resulting in a fidelity >90% for all chain lengths. The relative improvement is highest for low values of α , as seen in Fig. 3d . The C strategy outperforms the QAC strategy for sufficiently small chain lengths, but its performance drops quickly for large chain lengths. Furthermore, the crossover occurs at smaller chain lengths as the problem scale α is decreased. The NP strategy is competitive with QAC for relatively short chains but its performance also drops rapidly. The EP probability is initially intermediate between the U and (C, NP) cases, but always catches up with the (C, NP) data for sufficiently long chains and overtakes both for sufficiently small α . This shows that the EP strategy can be better than the purely classical strategies but by itself is insufficient, and it must be supplemented by decoding as in the complete QAC strategy. 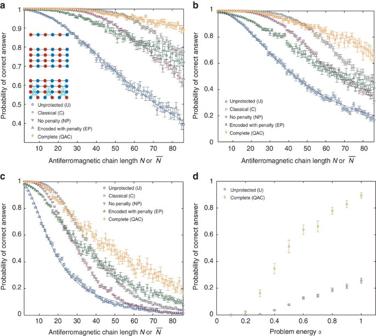Figure 3: Success probabilities of the different strategies. Panelsa–cshow the results for antiferromagnetic chains as a function of chain length forα=1, 0.6 and 0.3, respectively. At the largest chain lengths, the QAC strategy gives the largest success probability for all problem energy scalesα, showing significant improvements over all other strategies studied. The solid blue lines in the U case are best fits to 1/(1+qN2) (Lorentzian), yieldingq=1.94 × 10−4, 5.31 × 10−4, 3.41 × 10−3forα=1, 0.6 and 0.3, respectively. This rules out a simple classical thermalization process, which would predict an exponential decay withN(seeSupplementary Equation (2)inSupplementary Note 2). Paneldcompares the U and QAC strategies atN==86 andαε{0.1, 0.2, …, 1.0}. Chains shown inadepict the U (top), C (middle) and {NP, EP, QAC} (bottom) cases. In the bottom case, physical qubits of the same colour form an encoded qubit. Figure 3: Success probabilities of the different strategies. Panels a – c show the results for antiferromagnetic chains as a function of chain length for α =1, 0.6 and 0.3, respectively. At the largest chain lengths, the QAC strategy gives the largest success probability for all problem energy scales α , showing significant improvements over all other strategies studied. The solid blue lines in the U case are best fits to 1/(1+ qN 2 ) (Lorentzian), yielding q =1.94 × 10 −4 , 5.31 × 10 −4 , 3.41 × 10 −3 for α =1, 0.6 and 0.3, respectively. This rules out a simple classical thermalization process, which would predict an exponential decay with N (see Supplementary Equation (2) in Supplementary Note 2 ). Panel d compares the U and QAC strategies at N = =86 and α ε{0.1, 0.2, …, 1.0}. Chains shown in a depict the U (top), C (middle) and {NP, EP, QAC} (bottom) cases. In the bottom case, physical qubits of the same colour form an encoded qubit. Full size image Since α sets the overall problem energy scale, it is inversely related to the effective noise strength. This is clearly visible in Fig. 3a–d (see also Fig. 5 ), where the overall success probability improves significantly over a range of α values. The unprotected chains are reasonably well fit by a Lorentzian, whereas a classical model of independent errors (see Supplementary Note 2 ) fails to describe the data as it predicts an exponential dependence on N . Additional details, including from experiments on the D-Wave One ‘Rainier’ processor are given in Supplementary Note 1 . We turn next to an analysis and explanation of our results. Figure 5: Experimental optimization of the penalty strength β . 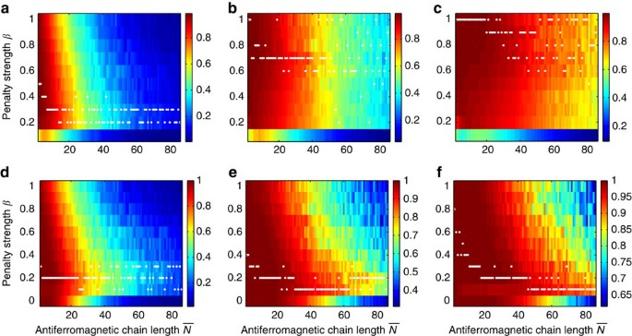Figure 5: Experimental optimization of the penalty strengthβ. The top (bottom) row shows colour density plots of the experimental success probability of the EP (QAC) strategy as a function ofβandε{2, 3, …, 86}, atα=0.3 (left), 0.6 (middle) and 1 (right). The optimalβvalues are indicated by the white dots. The optimalβvalues for the EP strategy are generally larger than that of the QAC strategy since the optimalβserves different purposes in these two cases. Note that atβ=0, where the QAC strategy becomes the NP strategy, we observe markedly lower success probability than at finiteβ, showing that a finite yet smallβfor large chain lengths is crucial to the QAC strategy. In contrast, the EP strategy performs poorly at very smallβas it does not recover probability lost to decodable states and requires a larger optimalβto increase the ground-state energy gap and reduce the error rate. The top (bottom) row shows colour density plots of the experimental success probability of the EP (QAC) strategy as a function of β and ε{2, 3, …, 86}, at α =0.3 (left), 0.6 (middle) and 1 (right). The optimal β values are indicated by the white dots. The optimal β values for the EP strategy are generally larger than that of the QAC strategy since the optimal β serves different purposes in these two cases. Note that at β =0, where the QAC strategy becomes the NP strategy, we observe markedly lower success probability than at finite β , showing that a finite yet small β for large chain lengths is crucial to the QAC strategy. In contrast, the EP strategy performs poorly at very small β as it does not recover probability lost to decodable states and requires a larger optimal β to increase the ground-state energy gap and reduce the error rate. Full size image Optimizing the penalty scale β To obtain the performance of the EP and QAC strategies shown in Fig. 3 , we optimized β separately for each strategy and for each setting of α and . To understand the role of β consider first how increasing β affects the size and position of the gap Δ. The excitations relevant to our error correction procedure are to the second excited state and above, since the ground state becomes degenerate at t f . In Fig. 4a we show that the relevant gap grows with increasing β , as desired. The gap position also shifts to the left, which is advantageous since it leaves less time for thermal excitations to act while the transverse field dominates. However, the role of β is more subtle than would be suggested by considering only the gap. When β << α the penalty has no effect, and when β ≫ α the penalty dominates the problem scale and the chains effectively comprise decoupled encoded qubits. Thus, there should be an optimal β for each ( , α) pair, which we denote as β opt . Without decoding we expect β opt ~ α based on the argument above, which is confirmed in Fig. 5 (upper panels). 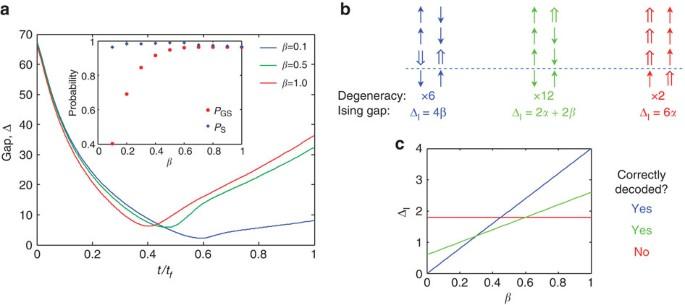Note that when β =0.1, the penalty is too small to be beneficial, and hence the poor performance for that value in the EP case. Figure 4: Effect of varying the penalty strengthβ. Panelashows the numerically calculated gap to the lowest relevant excited state for two antiferromagnetically coupled encoded qubits forα=0.3 and different values ofβ. Asβis increased, the minimum gap grows and moves to earlier in the evolution. Inset: undecoded (decoded) ground-state probabilityPGS(PS), where we observe a drop in the success probability beginning at approximatelyβ=0.6. Panelbshows three configurations of two antiferromagnetically coupled encoded qubits. Physical qubits denoted by heavy arrows point in the wrong direction. In the left configuration both encoded qubits have a bit-flip error, in the middle configuration only one encoded qubit has a single bit-flip error and in the right configuration one encoded qubit is completely flipped. The corresponding degeneracies and gaps (ΔI) from the final ground state are indicated, and the gaps plotted in panelc. The completely flipped (and undecodable) encoded qubit becomes the relevant excited energy state forβ≥0.6, which explains the drop in success probability observed in the simulations in panela. Therefore, the optimalβbalances the two key effects of increasing the gap and maintaining a majority of decodable states at low energies. Figure 4: Effect of varying the penalty strength β . Panel a shows the numerically calculated gap to the lowest relevant excited state for two antiferromagnetically coupled encoded qubits for α =0.3 and different values of β . As β is increased, the minimum gap grows and moves to earlier in the evolution. Inset: undecoded (decoded) ground-state probability P GS (P S ), where we observe a drop in the success probability beginning at approximately β =0.6. Panel b shows three configurations of two antiferromagnetically coupled encoded qubits. Physical qubits denoted by heavy arrows point in the wrong direction. In the left configuration both encoded qubits have a bit-flip error, in the middle configuration only one encoded qubit has a single bit-flip error and in the right configuration one encoded qubit is completely flipped. The corresponding degeneracies and gaps (Δ I ) from the final ground state are indicated, and the gaps plotted in panel c . The completely flipped (and undecodable) encoded qubit becomes the relevant excited energy state for β ≥0.6, which explains the drop in success probability observed in the simulations in panel a . Therefore, the optimal β balances the two key effects of increasing the gap and maintaining a majority of decodable states at low energies. Full size image In the QAC case another effect occurs: the spectrum is reordered so that undecodable states become lower in energy than decodable states. This is explained in Fig. 4b . Consider the three configurations shown. While the left and middle configurations are decodable, the right-side configuration is not. For sufficiently large α the undecodable state is always the highest of the three indicated excited states. The graph at the bottom of panel b shows the Ising gap as a function of β for α =0.3. While for sufficiently small β such that 4 β , 2 α +2 β <6 α both decodable states are lower in energy than the undecodable state, the undecodable state becomes the first excited state for sufficiently large β . This adversely affects the success probability after decoding, as is verified numerically in the inset of panel a, which shows the results of an adiabatic master equation [44] calculation for the same problem, yielding the undecoded ground-state probability P GS and the decoded ground-state probability P S (for model details and parameters, see the Methods section). While for β <0.6 decoding helps, this is no longer true when for β >0.6 the undecodable state becomes the first relevant excited state. Consequently, we again expect there to be an optimal value of β for the QAC strategy that differs from β opt for EP. These expectations are borne out in our experiments; Fig. 5 (lower panels) shows that β opt is significantly lower than in the EP case, which differs only via the absence of the decoding step. The decrease in β opt with increasing α and chain length can be understood in terms of domain wall errors (see below), which tend to flip entire encoded qubits, thus resulting in a growing number of undecodable errors. However, the benefit of even a small non-zero value for β opt at large chain lengths is critical in improving the outcome of the QAC strategy over the NP strategy as observed in Figs 3 and 5 , and can be viewed as indirect evidence of quantum effects. For additional insight into the roles of the penalty qubits α and β see Supplementary Notes 3 and 4 . Error mechanisms Solving for the ground state of an antiferromagnetic Ising chain is an ‘easy’ problem, so why do we observe decreasing success probabilities? As alluded to earlier, domain walls are the dominant form of errors for antiferromagnetic chains, and we show next how they account for the shrinking success probability. We analyse the errors on the problem versus the penalty qubits and their distribution along the chain. 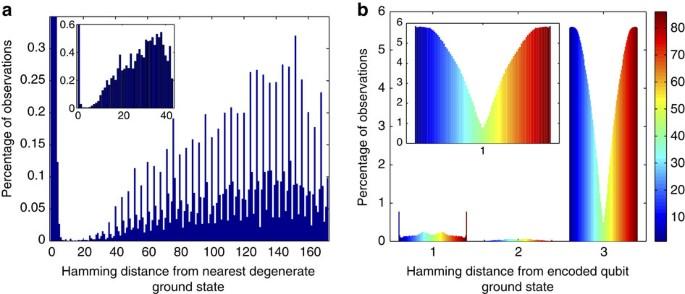Figure 6: Hamming distance histograms. Observed errors in encoded 86 qubit antiferromagnetic chains, atα=1 and the near-optimalβ=0.2. Panelais a histogram of Hamming distances from the nearest of the two degenerate ground states, measured in terms of physical qubits. The periodicity of four observed for Hamming distance ≥20 reflects the flipping of an entire encoded qubit. Inset: Hamming distance in terms of encoded qubits. The peaks at Hamming distance zero are cut off and extend to 63.6% (88.3%) for the physical (encoded) case. Panelbis a histogram of the errors as a function of encoded qubit position (colour scale) within the chain. Errors on encoded problem qubits are at Hamming distance 1, 2 or 3. Flipped penalty qubits are shown in the inset. The majority of errors are the flipping of entire encoded qubits (the flipped penalty qubits occur in conjunction with the flipping of all three problem qubits), corresponding to domain walls. Furthermore, errors occur predominantly at the chain boundaries, since errors cost half the energy there. The mirror symmetry is due to averaging over the two equivalent chain directions. Figure 6a is a histogram of the observed decoded states at a given Hamming distance d from the ground state of the =86 chains. The large peak near d =0 shows that most states are either correctly decoded or have just a few flipped bits. The quasi-periodic structure seen emerging at d ≥20 can be understood in terms of domain walls. The period is four, the number of physical qubits per encoded qubit, so this periodicity reflects the flipping of an integer multiple of encoded qubits, as in Fig. 4b . Once an entire encoded qubit has flipped and violates the antiferromagnetic coupling to, say, its left (thus creating a kink), it becomes energetically preferable for the nearest neighbour-encoded qubit to its right to flip as well, setting off a cascade of encoded qubit flips all the way to the end of the chain. The inset is the encoded Hamming distance histogram, which looks like a condensed version of the physical Hamming distance histogram because it is dominated by these domain wall dynamics. Figure 6: Hamming distance histograms. Observed errors in encoded 86 qubit antiferromagnetic chains, at α =1 and the near-optimal β =0.2. Panel a is a histogram of Hamming distances from the nearest of the two degenerate ground states, measured in terms of physical qubits. The periodicity of four observed for Hamming distance ≥20 reflects the flipping of an entire encoded qubit. Inset: Hamming distance in terms of encoded qubits. The peaks at Hamming distance zero are cut off and extend to 63.6% (88.3%) for the physical (encoded) case. Panel b is a histogram of the errors as a function of encoded qubit position (colour scale) within the chain. Errors on encoded problem qubits are at Hamming distance 1, 2 or 3. Flipped penalty qubits are shown in the inset. The majority of errors are the flipping of entire encoded qubits (the flipped penalty qubits occur in conjunction with the flipping of all three problem qubits), corresponding to domain walls. Furthermore, errors occur predominantly at the chain boundaries, since errors cost half the energy there. The mirror symmetry is due to averaging over the two equivalent chain directions. Full size image Rather than considering the entire final state, Fig. 6b integrates the data in Fig. 6a and displays the observed occurrence rates of the various classes of errors per encoded qubit in =86 chains. The histograms for one, two and three problem qubits flipping in each location are shown separately. The states shown at Hamming distance 1 in the histogram are decodable, and together represent the contribution of the majority vote decoding to the overall success probability (note that some errors have already been suppressed via the EP term, as shown in the EP series in Fig. 3 and discussed earlier in the text). Flipped penalty qubits are shown in the inset and are essentially perfectly correlated with d =3 errors, indicating that a penalty qubit flip will nearly always occur in conjunction with all problem qubits flipping as well. Thus, the penalty qubits function to lock the problem qubits into agreement, as they should (further analysis of the role of the penalty qubit in error suppression is presented in Supplementary Note 3 ). The overwhelming majority of errors are one or more domain walls between encoded qubits. The domains occur with higher probability the closer they are to the ends of the chain, since kink creation costs half the energy at the chain boundaries. The same low barrier to flipping a qubit at the chain ends also explains the large peaks at d =1. Our majority vote-decoding strategy correctly decodes errors with d =1, incorrectly decodes the much less frequent d =2 errors and is oblivious to the dominant d =3 domain wall errors, which present as logical errors. Therefore, the preponderance of domain wall errors at large is largely responsible for the drop seen in the QAC data in Fig. 3 . The two-qubit problem analysed in Fig. 4a,b suggests that logical errors can dominate the low-energy spectrum. We observe this phenomenon in Fig. 7 , which shows that decodable and undecodable states separate cleanly by Hamming distance but not by energy, with many high-energy states being decodable states. In this sense the problem of chains we are studying here is in fact unfavourable for our QAC scheme, and we might expect better performance for computationally hard problems involving frustration. 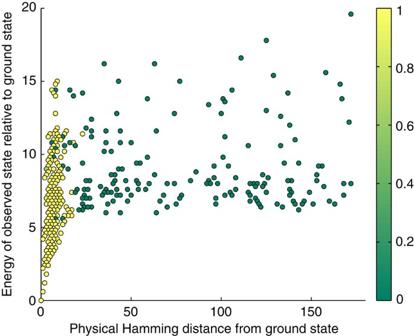Figure 7: Decodability analysis. The fraction of decodable states out of all states (colour scale) observed at a given Hamming distance from the nearest degenerate ground state (measured in physical qubits), and given energy above the ground state (in units ofJij=1), for=86 andα=1. Decodable states are observed predominantly at low Hamming distance and not necessarily at the lowest energy. Figure 7: Decodability analysis. The fraction of decodable states out of all states (colour scale) observed at a given Hamming distance from the nearest degenerate ground state (measured in physical qubits), and given energy above the ground state (in units of J ij =1), for =86 and α =1. Decodable states are observed predominantly at low Hamming distance and not necessarily at the lowest energy. Full size image Figure 7 lends itself to another interesting interpretation. Quantum annealing is normally understood as an optimization scheme that succeeds by evolving in the ground state, but how much does the energy of the final state matter when we implement error correction? Figure 7 shows that a small Hamming distance is much more strongly correlated with decodability than the final state energy: the latter can be quite high while the state remain decodable. Thus, the decoding strategy tolerates relatively high-energy final states. This work demonstrates that QAC can significantly improve the performance of programmable quantum annealing even for the relatively unfavourable problem of antiferromagnetic chains, which are dominated by encoded qubit errors manifested as domain walls. We have shown that increasing the problem energy scale by encoding into encoded qubits, introducing an optimum penalty strength β to penalize errors that do not commute with the penalty term, and decoding the excited states, reduces the overall error rate relative to any strategy that does less than these three steps, which comprise the complete QAC strategy. The next step is to extend QAC to problems where the correct solution is not known in advance, and is in fact the object of running the quantum annealer. Optimization of the decoding scheme would then be desirable. For example, detected errors could be corrected by solving a local optimization problem, whereby the values of a small cluster of encoded qubits that were flagged as erroneous and their neighbours are used to find the lowest energy solution possible. Other decoding schemes could be devised as needed, drawing, for example, on recent developments in optimal decoding of surface codes [50] . Another important venue for future studies is the development of more efficient QAC-compatible codes capable of handling larger weight errors. Ultimately, the scalability of quantum annealing depends on the incorporation of fault-tolerant error correction techniques, which we hope this work will help to inspire. Experiment details Most of our experiments were performed on the D-Wave Two (DW2) ‘Vesuvius’ processor at the Information Sciences Institute of the University of Southern California. The device has been described in detail elsewhere [32] , [51] , [52] . The D-Wave processors are organized into unit cells consisting of eight qubits arranged in a complete, balanced bipartite graph, with each side of the graph connecting to a neighbouring unit cell, as seen in Fig. 8 , known as the ‘Chimera’ graph [53] , [54] . The D-Wave One ‘Rainier’ processor is the predecessor of the DW2 and was used in our early experiments; it is described and compared with the DW2 in the Supplementary Method s and in Supplementary Note 1 . The annealing schedule for the DW2 is shown in Fig. 9 . 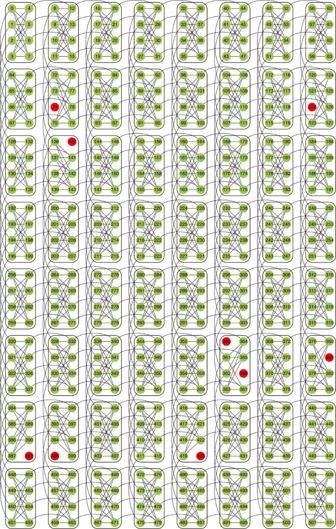Figure 8: Connectivity graph of DW2. The connectivity graph of the DW2 ‘Vesuvius’ processor consists of 8 × 8 unit cells of eight qubits (denoted by circles), connected by programmable inductive couplers (lines). The 503 green (red) circles denote functional (inactive) qubits. Most qubits connect to six other qubits. In the ideal case, where all qubits are functional and all couplers are present, one obtains the non-planar ‘Chimera’ connectivity graph. Figure 8: Connectivity graph of DW2. The connectivity graph of the DW2 ‘Vesuvius’ processor consists of 8 × 8 unit cells of eight qubits (denoted by circles), connected by programmable inductive couplers (lines). The 503 green (red) circles denote functional (inactive) qubits. Most qubits connect to six other qubits. In the ideal case, where all qubits are functional and all couplers are present, one obtains the non-planar ‘Chimera’ connectivity graph. 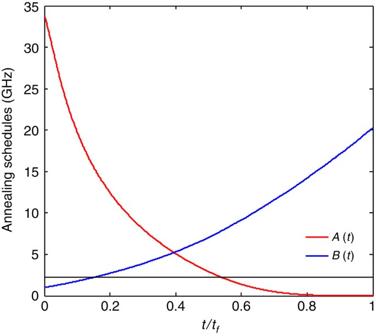Figure 9: DW2 annealing schedule. The functionsAandBare the ones appearing in equations (2) and (5). The solid horizontal black line is the operating temperature of 17mK. Full size image Figure 9: DW2 annealing schedule. The functions A and B are the ones appearing in equations (2) and (5). The solid horizontal black line is the operating temperature of 17mK. Full size image All our DW2 results were averaged over 24 embeddings of the chains on the processor (except U in Figs 2 and 3d , which used 188 embeddings), where an embedding assigns a specific set of physical qubits to a given chain. After programming the couplings, the DW2 device was cooled for 10 ms, and then 5,000 annealing runs per embedding were performed using the minimum DW2 annealing time of t f =20 μs for every problem size N , ε{2, 3,…, 86}, α ε{0.1, 0.2, ..., 1.0} and β ε{0.1, 0.2, ..., 1.0}. Annealing was performed at a temperature of 17 mK (≈2.2 GHz), with an initial transverse field starting at A (0)≈33.8 GHz, going to zero during the annealing, while the couplings are ramped up from near zero to B ( t f )≈20.5 GHz. Error bars Error bars in all our DW2 plots were calculated over the set of embeddings and express the s.e.m. σ / , where σ 2 = is the sample variance and S is the number of samples. Code and non-code states The ‘code states’ = and = of the encoded Ising Hamiltonian equation (3) are eigenstates of with eigenvalues n and − n , respectively. ‘Non-code states’ are the remaining 2 n −2 eigenstates, having at least one bit-flip error. The states and are eigenstates of , also with eigenvalues n and − n , respectively. Therefore, the ground state of is identical, in terms of the code states, to that of the original unencoded Ising Hamiltonian, with N = . Proof that the encoded graph is non-planar The solution of the Ising model over the encoded graph over the processor, shown in Fig. 1c is an NP-hard problem, just as the same problem over the original hardware graph is NP-hard. The key lies in the effectively three-dimensional nature of both graphs; the ground state of Ising spin glasses over non-planar lattices is an NP-hard problem [40] . We provide a graphical proof of non-planarity for the encoded graph here. The existence of a subgraph homeomorphic to the K 3,3 complete bipartite graph with three vertices on each side is sufficient to prove that a given graph is non-planar [55] . This subgraph may take as its edges paths within the graph being studied. We take a section of the encoded graph and, by performing a series of allowed moves of condensing paths to edges, show that the section is indeed homeomorphic to K 3,3 . We begin with an 18-qubit section of the regular encoded graph, shown in Fig. 10a . This encoded graph is then condensed along its paths by repeatedly removing two edges and a vertex and replacing them with a single edge representing the path. A clear sequence of these moves is shown in Fig. 10b–d . The studied subgraph has now been condensed into the form of the desired K 3,3 graph, as is made clear by labelling and rearranging the vertices as in Fig. 10e . The encoded graph is therefore proved non-planar. 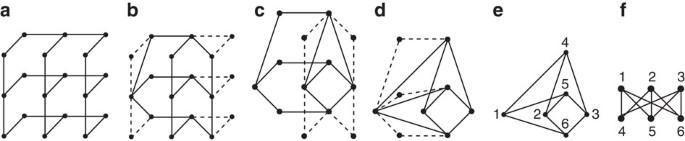Figure 10: Contraction of the encoded graph toK3,3. (a) A portion of the encoded graph over encoded qubits. (b–d) Contraction of paths in the original graph into edges. Paths consisting of two edges and a vertex are selected (represented in the figure as dotted lines), and then contracted into a single edge connecting the ends of the chosen path (shown as a new solid line). The condensed graph (e) is isomorphic to the standard representation of theK3,3bipartite graph (f). Figure 10: Contraction of the encoded graph to K 3,3 . ( a ) A portion of the encoded graph over encoded qubits. ( b – d ) Contraction of paths in the original graph into edges. Paths consisting of two edges and a vertex are selected (represented in the figure as dotted lines), and then contracted into a single edge connecting the ends of the chosen path (shown as a new solid line). The condensed graph ( e ) is isomorphic to the standard representation of the K 3,3 bipartite graph ( f ). Full size image Adiabatic Markovian master equation To derive the master equation used in performing the simulations, we consider a closed system with Hamiltonian where H S ( t ) is the time-dependent system Hamiltonian (which in our case takes the form given in equation (2)), H B is the bath Hamiltonian, { A α } are Hermitian system operators, { B α } are Hermitian bath operators and g is the system–bath interaction strength (with dimensions of energy). Under suitable approximations, a master equation can be derived from first principles [44] describing the Markovian evolution of the system. This equation takes the Lindblad form [56] : where H LS is the Lamb shift term induced by the interaction with the thermal bath, ω is a frequency, γ αβ ( ω ) is a positive matrix for all values of ω and L α,ω ( t ) are time-dependent Lindblad operators. They are given by where is the Cauchy principal value, Δ ba ( t )≡ ε b ( t )− ε a ( t ), and the states | ε a ( t )〉 are the instantaneous energy eigenstates of H S ( t ) with eigenvalues ε a ( t ) satisfying For our simulations, we considered independent dephasing harmonic oscillator baths (that is, each qubit is coupled to its own thermal bath) such that where b k , α and are, respectively, lowering and raising operators for the k th oscillator of the bath associated with qubit α and satisfying [ b k , α , ]= δ k , k ′ for all α . Furthermore, we assume an Ohmic spectrum for each bath such that where β is the inverse temperature, η (with units of time squared) characterizes the Ohmic bath and ω c is a UV cutoff. In our simulations, we fix ω c =8π GHz to satisfy the approximations made in deriving the master equation (see Albash et al. [44] for more details), and we fix β −1 /≈2.2 GHz to match the operating temperature of 17 mK of the D-Wave device. The only remaining free parameter is the effective system–bath coupling that we vary to find the best agreement with our experimental data. Further details are given in Supplementary Note 2 . How to cite this article: Pudenz, K. L. et al. Error-corrected quantum annealing with hundreds of qubits. Nat. Commun. 5:3243 doi: 10.1038/ncomms4243 (2014).